Carrier-envelope phase-dependent high harmonic generation in the water window using few-cycle infrared pulses High harmonic generation (HHG) using waveform-controlled, few-cycle pulses from Ti:sapphire lasers has opened emerging researches in strong-field and attosecond physics. However, the maximum photon energy of attosecond pulses via HHG remains limited to the extreme ultraviolet region. Long-wavelength light sources with carrier-envelope phase stabilization are promising to extend the photon energy of attosecond pulses into the soft X-ray region. Here we demonstrate carrier-envelope phase-dependent HHG in the water window using sub-two-cycle optical pulses at 1,600 nm. Experimental and simulated results indicate the confinement of soft X-ray emission in a single recombination event with a bandwidth of 75 eV around the carbon K edge. Control of high harmonics by the waveform of few-cycle infrared pulses is a key milestone to generate soft X-ray attosecond pulses. We measure a dependence of half-cycle bursts on the gas pressure, which indicates subcycle deformation of the waveform of the infrared drive pulses in the HHG process. Waveform-controlled, few-cycle optical pulses from Ti:sapphire lasers have opened the opportunity to explore electric-field-sensitive strong-field experiments and to generate attosecond pulses for spectroscopic applications [1] . However, the maximum photon energy of isolated attosecond pulses via high harmonic generation (HHG) using an 800-nm electric field has been limited in the extreme ultraviolet (EUV; <200 eV) because of the cutoff law in HHG [2] . To extend the spectral range of high harmonics (HHs) from the EUV to the soft X-ray region, long-wavelength light sources are promising candidates. This contradictory argument can be explained with a semi-classical three-step model [2] . The first step is tunnelling ionization at the peak of a strong electric field, which releases an electron wavepacket into the continuum from an atom. In the second step, the wavepacket is accelerated by the field and gains substantial kinetic energy. In the final step, the wavepacket is driven back to the vicinity of the parent ion by the reversed electric field and recombines with it, emitting a photon of energy equal to the sum of the kinetic energy and the ionization potential. The highest possible photon energy within this framework is called as the cutoff energy, and it is given by E cutoff = I p +3.17 U p , where I p is the ionization potential of a target atom, U p [eV]=9.3 × 10 −14 I (W cm −2 ) × ( λ (μm)) 2 is the ponderomotive energy, and I and λ are the laser intensity and wavelength, respectively. The maximum intensity applicable to a target medium is limited by the saturation of its ionization, which shows no dependence on the centre wavelength of the electric field and small dependence on its temporal duration. Thus, it is evident that the cutoff energy can be significantly extended using a long-wavelength electric field because of the square dependence of U p on λ . Pioneering HHG experiments have demonstrated the usability of infrared pulses to extend the cutoffs [3] , [4] . Furthermore, recent experiments using multi-millijoule pulses from infrared or mid-infrared optical parametric amplifiers (OPAs) have achieved drastic extension of the cutoff to the water window [5] and even to more than 1 keV (Popmintchev et al. [6] ). These experiments have used relatively long femtosecond infrared pulses without controlling a carrier-envelope phase (CEP). As a result, the temporal resolution obtained with such HHs is generally limited by the envelope of the drive pulses and remains on a femtosecond time scale. Stabilization of the CEP of few-cycle pulses is essential to trigger the dynamics of a quantum system with subcycle accuracy and, therefore, with attosecond temporal resolution. Recent success in attosecond physics has exclusively owed to CEP-stabilized, few-cycle optical pulses at ~800 nm based on Ti:sapphire laser technologies [7] , [8] , [9] , [10] . Progress in frequency conversion of optical pulses based on either broadband OPAs or optical parametric chirped-pulse amplifiers (OPCPAs) has realized the generation and amplification of few-cycle intense pulses in the infrared with CEP stabilization [11] , [12] , [13] . Such high-energy infrared light sources have been applied to the extension of the HH cutoffs [14] , [15] , [16] up to 200 eV. However, a CEP dependence of soft X-ray harmonics, particularly beyond the carbon K edge, has not been demonstrated. We have developed an OPCPA using BiB 3 O 6 (BIBO) crystals pumped by a Ti:sapphire laser [17] . BIBO-based OPAs or OPCPAs possess an extremely broadband gain spectrum, which extends nearly one octave (1,200–2,200 nm) under a collinear phase-matching condition at degeneracy when pump lasers at 800 nm are used [18] , [19] . In a BIBO-OPCPA, few-cycle, intense infrared pulses can be directly generated from the amplifier without nonlinear spectral broadening. The output pulses from our BIBO-OPCPA have extremely good shot-to-shot stability both in the output energy and the CEP: 0.85% (root mean square; r.m.s.) and 160 mrad (r.m.s. ), respectively [17] . The long-term drifts of the output energy and the CEP are also measured to be better than 2% and 100 mrad over 24 h, respectively. In this work, we generate HHs from neon, which exhibit spectral extension to the water window with a clear dependence on the CEP of the sub-two-cycle infrared pulses from the OPCPA. The observed CEP dependence is well reproduced by simulation results based on the strong-field approximation (SFA) [20] and shows a clear separation of the spectra of half-cycle soft X-ray bursts. Our experimental and simulated results indicate the confinement of soft X-ray emission in a single recombination event, which has a bandwidth of 75 eV around the carbon K edge. We also observe that the cutoffs of half-cycle bursts respond differently to the backing pressure of the neon gas, which reveals subcycle nonlinear deformation of the few-cycle infrared pulses in the HHG process. HHG in the water window We used optical pulses at a wavelength of 1,600 nm and a repetition rate of 1 kHz from the infrared OPCPA ( Fig. 1a ) for HHG experiments. This light source is capable of delivering 9.0 fs, 550 μJ, CEP-stabilized optical pulses. 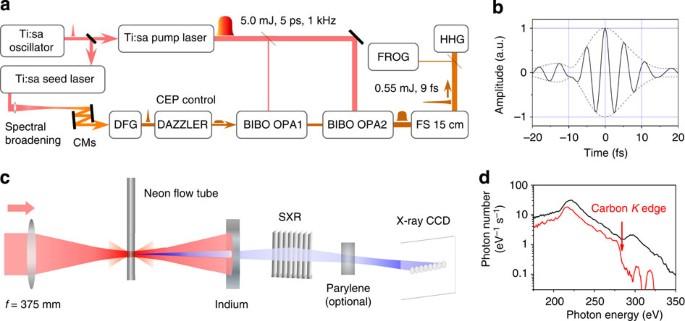Figure 1: Experimental set-up. (a) Schematic of the IR OPCPA system. Difference frequency generation (DFG) crystal for CEP-stabilized seed pulses; DAZZLER acousto-optic programmable dispersive filter (Dazzler, FASTLITE); BIBO OPA 1 and OPA2, first and second BIBO OPA stages, respectively; FS, 150-mm-long glass block made of synthetic fused silica; FROG, frequency-resolved optical gating apparatus; HHG, high harmonic generation set-up. (b) Electric field of the 1,600-nm, 9.0-fs optical pulses with acos-like waveform (solid line) and its envelope (dashed lines). (c) Set-up for the generation of soft X-ray HHs detected by the X-ray charge-coupled device camera after the soft X-ray spectrometer (SXR). A 150-nm-thick indium filter is inserted to block the fundamental beam and low-order harmonics below 140 eV. (d) HH spectra recorded with (red line) and without (black line) two 200-nm-thick parylene filters. The sharp intensity drop indicates the absorption of the carbonKedge at 284 eV by the parylene filters. Figure 1b shows an example of the cos -like waveform of the 9.0 fs infrared pulses, which were characterized by frequency-resolved optical gating. The OPCPA output beam was focused by a spherical mirror with a focal length of 375 mm into a 1.4-mm-thick gas cell filled with neon set in a vacuum chamber ( Fig. 1c ). The backing pressure of the cell was varied up to 1.4 atm. The pulse energy of the infrared beam was adjusted to be 380 μJ using a diaphragm with a 20-mm-diameter aperture for all the measurements in this work. The fundamental beam and low-order harmonics below ~140 eV were blocked by a 150-nm-thick indium filter, which was placed in front of a soft X-ray spectrometer (SXR-II-1, Hettrick Scientific). Spectrally resolved HHs were detected by a back-illuminated X-ray charge-coupled device camera (PIXIS-XO-2048B, Princeton Instruments). The exposure time of the camera was set to be 10 s. The red and black lines of Fig. 1d plot HH spectra that were recorded with and without two additional 200-nm-thick parylene filters, respectively. The sharp intensity drop at 284 eV of the red line is due to the absorption of the carbon K edge. Intensity distributions of harmonic spectra are plotted by the photon flux (photon number per eV per second) in front of the camera after intensity calibration. Figure 1: Experimental set-up. ( a ) Schematic of the IR OPCPA system. Difference frequency generation (DFG) crystal for CEP-stabilized seed pulses; DAZZLER acousto-optic programmable dispersive filter (Dazzler, FASTLITE); BIBO OPA 1 and OPA2, first and second BIBO OPA stages, respectively; FS, 150-mm-long glass block made of synthetic fused silica; FROG, frequency-resolved optical gating apparatus; HHG, high harmonic generation set-up. ( b ) Electric field of the 1,600-nm, 9.0-fs optical pulses with a cos -like waveform (solid line) and its envelope (dashed lines). ( c ) Set-up for the generation of soft X-ray HHs detected by the X-ray charge-coupled device camera after the soft X-ray spectrometer (SXR). A 150-nm-thick indium filter is inserted to block the fundamental beam and low-order harmonics below 140 eV. ( d ) HH spectra recorded with (red line) and without (black line) two 200-nm-thick parylene filters. The sharp intensity drop indicates the absorption of the carbon K edge at 284 eV by the parylene filters. Full size image CEP-dependent half-cycle cutoffs A relative CEP, Δ φ CEP , of the infrared pulses was scanned by an acousto-optic programmable dispersive filter (Dazzler, HR45-1200-2200, FASTLITE). Note that Δ φ CEP is a relative value, of which the phase offset was adjusted to match experimental data with simulated results. 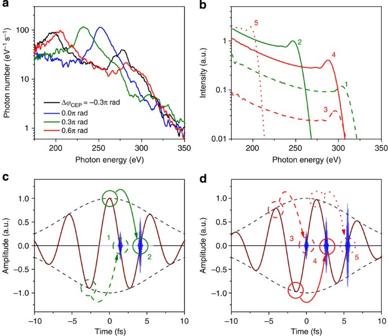Figure 2: CEP-dependent HCOs associated with the electron trajectories in a sub-two-cycle pulse. (a) Four HH spectra recorded at ΔφCEPs in steps of 0.3π rad. The spectra contain one or two peaks, which are attributed to the HCOs of harmonic emissions from two major electron trajectories. (b) Spectral distributions of soft X-ray emissions, which are calculated by an SFA-based simulation assuming 10-fs optical pulses at 1,600 nm with an intensity of 3.8 × 1014W cm−2. Each burst is filtered out by a temporal gate to select dipole emission contributed from the short trajectory. The duration of the gate was set to be approximately one-third of the oscillation period of a 1,600-nm field (~1.8 fs). The green dashed and solid curves plot the spectral distributions of dipole emissions under thecos-like waveform, which result from the electron trajectories represented by the dashed and solid curves in Fig. 2c, respectively. The red dashed, solid and dotted curves plot the spectral distributions of dipole emissions under thesin-like waveform, which result from the electron trajectories represented by the dashed, solid and dotted curves in Fig. 2d, respectively. (c,d) Dominant electron trajectories under thecos-like andsin-like waveforms, respectively. The spectral distributions of electric dipoles are shown in Fig. 2b. The numbers and the colours associated with the electron trajectories are matched with Fig. 2b. Figure 2a shows HH spectra that were recorded at four CEPs in steps of 0.3π rad. We found that one or two peaks in the HH spectra were drastically shifted by the change of the CEP at a rate of 75 eV (π rad) −1 . These peaks are attributed to be half-cycle cutoffs (HCOs) that originate from several electron trajectories allowed in a few-cycle pulse-driven HHG process [21] . The spectral density of each dipole emission increases near the cutoff, which results in the spectral peaks. Such spectral structures have been observed both theoretically [2] and experimentally [21] . To understand the behaviour of the observed HCOs, we simulate the spectra of half-cycle bursts using the SFA. We consider an HHG process with two CEPs of a sub-two-cycle pulse as shown in Fig. 2c,d . These figures depict electron trajectories that are mainly allowed under the cos - and sin -like waveforms, respectively. Figure 2b represents the spectral distributions of electric dipoles as a result of the electron trajectories that are shown in Fig. 2c,d . Parameters used in the simulations are listed in the caption of Fig. 2 . Shifting the CEP of a few-cycle field significantly changes the amplitude of each half cycle. Therefore, the cutoff energy of soft X-ray emission from each trajectory exhibits a dependence on the CEP. The sum of the spectra of the individual bursts in Fig. 2b well reproduces the experimental HH spectra in Fig. 2a . The experimental and the simulated HH spectra are quantitatively consistent in (i) the positions of the HCOs, (ii) the amount of the energy shift of the HCOs with respect to the CEP, and (iii) the intensity ratio between the two HCOs. The highest HCO reaches to ~325 eV as shown by the green line in Fig. 2a . This cutoff energy is consistent with previous works [6] , [22] . Figure 2: CEP-dependent HCOs associated with the electron trajectories in a sub-two-cycle pulse. ( a ) Four HH spectra recorded at Δ φ CEP s in steps of 0.3π rad. The spectra contain one or two peaks, which are attributed to the HCOs of harmonic emissions from two major electron trajectories. ( b ) Spectral distributions of soft X-ray emissions, which are calculated by an SFA-based simulation assuming 10-fs optical pulses at 1,600 nm with an intensity of 3.8 × 10 14 W cm −2 . Each burst is filtered out by a temporal gate to select dipole emission contributed from the short trajectory. The duration of the gate was set to be approximately one-third of the oscillation period of a 1,600-nm field (~1.8 fs). The green dashed and solid curves plot the spectral distributions of dipole emissions under the cos -like waveform, which result from the electron trajectories represented by the dashed and solid curves in Fig. 2c, respectively. The red dashed, solid and dotted curves plot the spectral distributions of dipole emissions under the sin -like waveform, which result from the electron trajectories represented by the dashed, solid and dotted curves in Fig. 2d, respectively. ( c , d ) Dominant electron trajectories under the cos -like and sin -like waveforms, respectively. The spectral distributions of electric dipoles are shown in Fig. 2b. The numbers and the colours associated with the electron trajectories are matched with Fig. 2b. Full size image We measured a collection of CEP-dependent HH spectra ( Fig. 3a ) that were recorded in steps of 0.1π rad. The backing pressure of neon was set at 0.6 atm. The HH spectra were reproduced every π rad of the CEP. This observation is a consequence of the HHG process because a CEP shift by π rad spatially inverts the electric field of drive pulses, which does not affect the spectral intensity of HHs. The SFA-based simulation in Fig. 3b has been conducted to reproduce the observed CEP dependence. The best match to the experimental data is found by assuming a pulse duration of 10 fs (FWHM of intensity), a peak intensity of 3.8 × 10 14 W cm −2 and a centre wavelength of 1,600 nm. Here the experimental CEP values have an ambiguity of π rad. The spectra of calculated dipoles contain modulated structures from interference among the two emissions from the short and long electron trajectories in a single recombination event. The emission from the latter is usually suppressed under appropriate phase-matching conditions [23] . The soft X-ray continuum generated in a single recombination event when Δ φ CEP =−0.3π rad as shown in Figs 2a and 3a has the maximum bandwidth of ~75 eV around the carbon K edge. When higher laser intensity was applied onto the gas target, peak structures and CEP dependence in the HH spectra disappeared. This behaviour is most probably due to heavy ionization and associated plasma effects, which degrade the phase coherence of generated HHs. Such observation for HH spectra around 180 eV has been demonstrated using near-infrared drive pulses at 800 nm (Ishii et al. [24] ). 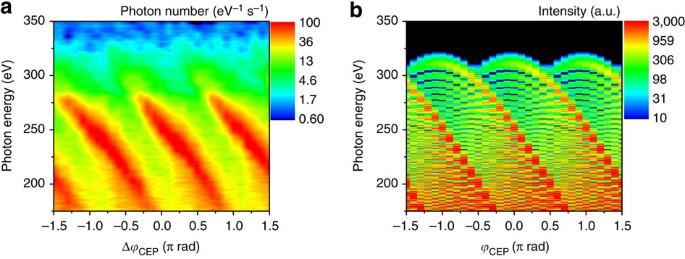Figure 3: CEP-dependent HH spectra. (a) Experimentally obtained HH spectra recorded at ΔφCEPs in steps of 0.1π rad and at a backing pressure of 0.6 atm. (b) Simulated HH spectra assuming 10 fs optical pulses at 1,600 nm with an intensity of 3.8 × 1014W cm−2. Figure 3: CEP-dependent HH spectra. ( a ) Experimentally obtained HH spectra recorded at Δ φ CEP s in steps of 0.1π rad and at a backing pressure of 0.6 atm. ( b ) Simulated HH spectra assuming 10 fs optical pulses at 1,600 nm with an intensity of 3.8 × 10 14 W cm −2 . Full size image Pressure dependence of HCOs In the next experiment, we investigated the dependence of the HCOs on the target gas pressure. This experiment was carried out in the same run with the equivalent parameters as those used in the previous measurement. The peak power of the infrared pulses was 38 GW, which is approximately two times more than the critical power of 21 GW for self-focusing when the pressure of neon is set at 1.0 atm (Börzsönyi et al. [25] ). 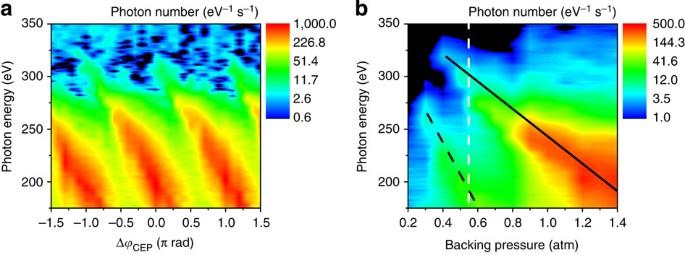Figure 4: CEP and pressure dependences of HH spectra. (a) Experimentally obtained HH spectra recorded at ΔφCEPs in steps of 0.1π rad and at a backing pressure of 1.0 atm. (b) Pressure dependence of HH spectra. The black solid and dashed lines are drawn along the spectral peaks that originate from different HCOs. The white dashed line is drawn at the gas pressure of the self-focusing threshold (0.55 atm) when the critical power is identical to the peak power of the infrared pulses (38 GW). Figure 4a shows the CEP dependence of soft X-ray spectra measured at a backing pressure of 1.0 atm. By increasing the backing pressure from 0.6 to 1.0 atm, on-axis intensities of HHs below 280 eV increased by nearly one order of magnitude. The conversion efficiency from the infrared pulse to the soft X-ray continuum in the photon energy range between 150 and 300 eV is calculated to be on the order of 10 −9 after the spectrometer, which is consistent with HHG experiments that use 800 nm drive pulses by taking the wavelength scaling of λ −(5–6) into account [26] , [27] , [28] . The CEP-dependent HH spectra at 1.0 atm show a similarity to that observed with a backing pressure of 0.6 atm. However, the spectral widths of the half-cycle bursts were broadened and their locations were shifted horizontally by −(0.3–0.5)π rad depending on the photon energies. We presume that such spectral dependences of the peak shift are caused by subcycle deformation of the waveform of the infrared pulses. Figure 4: CEP and pressure dependences of HH spectra. ( a ) Experimentally obtained HH spectra recorded at Δ φ CEP s in steps of 0.1π rad and at a backing pressure of 1.0 atm. ( b ) Pressure dependence of HH spectra. The black solid and dashed lines are drawn along the spectral peaks that originate from different HCOs. The white dashed line is drawn at the gas pressure of the self-focusing threshold (0.55 atm) when the critical power is identical to the peak power of the infrared pulses (38 GW). Full size image We scanned the backing pressure from 0.2 to 1.4 atm with a fixed CEP (Δ φ CEP =−0.3π rad) to examine responses of the HCOs. The pressure at the interaction region is estimated to be on the same order as the backing pressure of the gas cell because of low conductance through two tiny holes (diameter <100 μm), which were drilled by the infrared beam. Figure 4b plots the pressure dependence of the HCOs. By increasing the pressure from 0.2 to 0.4 atm, the on-axis intensity of HHs rapidly increased, which indicates the onset of self-guiding of the infrared pulses [6] . The HH spectrum at 0.6 atm in Fig. 4b contains two HCOs located at ~180 and 280 eV. These two HCOs were shifted downwards with different slopes when the gas pressure was increased. The lower-energy peak downshifts with a slope of −280 eV atm −1 (indicated by the black dashed line in Fig. 4b ), whereas the higher-energy peak downshifts with a slope of −130 eV atm −1 (the black solid line in Fig. 4b ). This fact also supports the above-mentioned mechanism of waveform deformation induced by cycle-dependent phase modulation by nonlinear processes such as self-phase modulation, self-focusing and plasma effects. From these dependences, we can obtain information about cycle-dependent nonlinear interactions between the driver electric field and a gaseous medium. Subcycle deformation of a driver laser field has been theoretically investigated [29] , [30] , [31] , and also discussed to explain the spectral shift of HH combs [32] , [33] , [34] . In our case, a two-dimensional plot can be used to reveal a pressure dependence of HCOs originated from consecutive electron trajectories as clear evidence of waveform deformation. The CEP dependences in Figs 3a and 4a also indicate that pressure-induced deformation upshifts the instantaneous frequency of the subcycle waveform. Such frequency upshift causes the reduction of the HCOs and the increase of the slope that traces the spectral peaks at the HCOs in Fig. 4a compared with Fig. 3a . A CEP dependence of HHs using few-cycle Ti:sapphire lasers at 800 nm has usually been observed as spectral transition around the cutoff of the HHs from modulated structures to the appearance of a continuum in the EUV [7] . This method must spectrally resolve adjacent harmonic combs that are separated by twice the photon energy of Ti:sapphire laser pulses. For 1,600 nm drive pulses, this method requires a spectral resolution of a fraction of 1.5 eV around 300 eV, which is difficult to achieve with a compact soft X-ray spectrometer. Recent observation of CEP dependences using HCOs in the EUV has been used to experimentally determine the CEP of few-cycle Ti:sapphire laser pulses [21] . In this work, we have shown the dependence of the HCOs on the CEP of the few-cycle infrared pulses to determine the CEP value of the drive pulses. Our experimental and simulated results indicate, at a certain CEP value, the confinement of soft X-ray emission into a single recombination event near the cutoff, which has a 75-eV-wide bandwidth around the carbon K edge. A wide continuum generated by a long-wavelength driver is more advantageous than that generated by Ti:sapphire lasers for potential generation of shorter attosecond pulses. To date, researchers have attained the shortest attosecond pulses with a sub-two-cycle temporal duration of 67 as in the EUV [35] . Further shortening of attosecond pulses requires longer-wavelength drivers to upshift their frequency to the soft X-ray region. In conclusion, we applied the infrared light source based on the BIBO-OPCPA scheme to generate HHs in the water window that exhibit the clear dependence on the CEP of the sub-two-cycle infrared pulses. The highest HCO reaches 325 eV, which is well beyond the carbon K edge. The experimental observations such as the spectral structures and CEP dependences of the half-cycle bursts are well reproduced by the SFA-based simulated results assuming 10 fs, 1,600 nm optical pulses with an intensity of 3.8 × 10 14 W cm −2 . The HH spectra consist of a few peaks located at different spectral positions; these peaks are attributed to the HCOs that originate from electron trajectories allowed in the few-cycle pulse-driven HHG process. The experimental and simulated results indicate the confinement of soft X-ray emission in a single recombination event, which has a bandwidth of ~75 eV around the carbon K edge. This work shows the general capability of CEP-stable few-cycle intense infrared pulses towards generation of isolated coherent soft X-ray pulses and their applications to ultrafast soft X-ray spectroscopy with a temporal resolution from attoseconds to few femtoseconds. Infrared OPCPA system Here we describe the details of the infrared OPCPA system. Readers are also referred to elsewhere [18] . A schematic of the OPCPA is presented in Fig. 1 . The output pulses from a Ti:sapphire oscillator seeded two Ti:sapphire chirped-pulse amplification (CPA) systems where one system was used to produce infrared seed pulses, and the other to pump BIBO-OPAs. Femtosecond output pulses from one of the two CPA systems is focused into a 1.6-bar krypton gas cell for spectral broadening via filamentation. Infrared seed pulses were produced by difference frequency generation between the blue and red spectral components of the broadened spectrum. The generated seed pulses, which carry a stabilized CEP owing to the difference frequency generation process, were temporally stretched to about 4 ps in the acousto-optic programmable dispersive filter. We obtained 5 mJ, 5 ps OPA pump pulses at 1 kHz and 805 nm from the other CPA system. The infrared seed pulses were amplified in two OPA stages, which consisted of 4-mm-thick and 6-mm-thick BIBO crystals both cut at θ =11.4° for type I interaction in the xz plane, respectively. The output energy after the first stage was typically 10 μJ using 0.2-mJ pump pulses. We achieved an output energy of 550 μJ after the second OPA with a conversion efficiency of 12%. We obtained nearly an octave gain bandwidth from 1,200 to 2,200 nm. Shot-to-shot energy fluctuations of the output pulses were measured to be 0.85% (r.m.s.). The amplified pulses were then compressed in a 150-mm-long glass block made of synthetic fused silica (SK1310, Ohara quartz). The compressed pulses were characterized by a third-harmonic generation-based frequency-resolved optical gating apparatus to have a duration of 9.0 fs (FWHM), which contains a 1.7-cycle electric field at 1,600 nm. The CEP stability of the amplified pulses was measured in a single-shot f -to- 2f interferometer to be 160 mrad. HHG chamber and spectrometer The output beam from the OPCPA was focused into a 1.4-mm-thick gas cell filled with neon in the vacuum chamber ( Fig. 1c ). The backing pressure of the cell was limited up to 1.4 atm by the capacity of a turbomolecular pump (STP-A803C, Edwards) attached to the chamber. The HHG chamber was maintained at 2.8 × 10 −2 Pa when the backing pressure was set at 0.6 atm, and the flow rate of neon was 40 sccm. Generated harmonics were spectrally dispersed by the soft X-ray spectrometer. This spectrometer images the source point of HHs to the charge-coupled device camera while HHs are spectrally resolved in one dimension. The spectrometer has been calibrated using parylene and boron filters to identify the K edges of carbon at 284 eV and boron at 188 eV, respectively. How to cite this article: Ishii, N. et al. Carrier-envelope phase-dependent high harmonic generation in the water window using few-cycle infrared pulses. Nat. Commun. 5:3331 doi: 10.1038/ncomms4331 (2014).